Design principle for increasing charge mobility of π-conjugated polymers using regularly localized molecular orbitals The feasibility of using π-conjugated polymers as next-generation electronic materials is extensively studied; however, their charge mobilities are lower than those of inorganic materials. Here we demonstrate a new design principle for increasing the intramolecular charge mobility of π-conjugated polymers by covering the π-conjugated chain with macrocycles and regularly localizing π-molecular orbitals to realize an ideal orbital alignment for charge hopping. Based on theoretical predictions, insulated wires containing meta -junctioned poly(phenylene–ethynylene) as the backbone units were designed and synthesized. The zigzag wires exhibited higher intramolecular charge mobility than the corresponding linear wires. When the length of the linear region of the zigzag wires was increased to 10 phenylene–ethynylene units, the intramolecular charge mobility increased to 8.5 cm 2 V −1 s −1 . Theoretical analysis confirmed that this design principle is suitable for obtaining ideal charge mobilities in π-conjugated polymer chains and that it provides the most effective pathways for inter-site hopping processes. Inorganic semiconductor materials are important for fabricating nanoscale electronic devices that are fundamental to the modern information society. Although new materials are constantly emerging, silicon has remained the semiconductor material of choice. However, π-conjugated organic materials, in particular π-conjugated polymers, are expected to be the next generation of monomolecular electronic materials [1] , [2] , [3] for molecular devices [4] , [5] , [6] , [7] , [8] because, despite their current poor stability, they have many advantages over silicon-based semiconductor materials, such as flexibility, light-weight and processability. The most serious problem associated with the development of π-conjugated polymers as electronic materials is that their charge mobility—the most dominant factor affecting carrier transport ability, and therefore, the most important property of semiconductors—is not comparable to that of silicon-based semiconductor materials. In an effort to overcome this challenge, we have successfully developed chemically stable insulated molecular wires (IMWs) with high charge mobilities (0.5–0.7 cm 2 V −1 s −1 ) (refs 9 , 10 , 11 , 12 ) comparable to those of amorphous silicon (1–10 cm 2 V −1 s −1 ), even in solid films. These materials were developed by covering π-conjugated polymers with cyclic molecules to isolate the polymer chains [13] , [14] , [15] and realize carrier hopping within them. This approach is more effective than the intermolecular carrier hopping predominantly observed during charge transfer in common π-conjugated organic materials. For the optimization of charge carrier mobility in the band-conduction (coherent charge carrier transport) regime, tightly locked polymer backbones with widespread π-conjugated planes have been successfully developed, giving high charge carrier mobility of over 500 cm 2 V −1 s −1 (ref. 16 ). This implies that further extension of the conjugated molecular plane will lead to the ultrahigh charge carrier mobility observed in perfect two-dimensional graphene [17] . Unlike the approach involving simple extension of conjugated molecular systems from one dimension to two dimensions, the potential of a ‘real’ one-dimensional conjugated backbone is revealed as a platform for the complete hopping transport of charge carriers in this study. We envisioned the possibility of further improving the intramolecular mobility of charge carrier hopping by localizing the π-conjugated chains at regular points to equalize the distance and molecular orbital levels between the hopping sites. This method was hypothesized to induce more effective internal carrier hopping, which is the rate-determining step in the charge transfer process for insulated π-conjugated polymer chains. In π-conjugated molecules, orbital delocalization over the planar region is quite effective for obtaining high charge mobility, because the delocalized orbitals provide the ideal pathways for coherent charge transport. However, the delocalization is easily disturbed by the thermally activated structural fluctuation/deformation that occurs in most long π-conjugated molecules, particularly polymers, but not carbon nanotubes or graphene derivatives. Thus, at ambient temperature, the charge transport in π-conjugated polymers can no longer be described by the electronic band picture because the structural deformation results in the localization of the π-orbitals and in turn charge hopping processes become dominant. Because the orbital energies of the localized π-orbitals depend on the area of localization, uncontrolled structural deformations will result in widely distributed orbitals (that is, wide density of states (DOS)) over a given energy range ( Fig. 1a ), which is not suitable for efficient charge hopping. Therefore, a narrow distribution of π-orbital levels (that is, narrow DOS) is the key condition for the efficient charge hopping in π-conjugated polymers ( Fig. 1b ). To realize this situation, we adopted oligo(phenylene–ethynylene) (OPE) as test oligomers ( Fig. 1c ), and introduced meta -junctions ( Fig. 1d ) to regularly break the orbital delocalization at the joint positions [18] , leading to regularly localized orbitals (see Supplementary Notes 1 and 2 for the orbital localizations by the meta -junctions). It can be seen that the narrow DOS can be realized in the meta -system by observing the π-orbitals at ambient temperature, where the benzene fragments can rotate almost freely (that is, a structural deformation). Considering the perpendicularly rotated benzenes at position 1 (1′), 2 (2′) or 3 (3′) and at those combinations in the seven benzene unit shown in Fig. 1c , six and four levels of localized π-orbitals are obtained in the para - and meta -junctioned systems, respectively, and the energetically higher orbitals, E 5 and E 6 , do not appear in the meta -system ( Fig. 1e ). Note that orbitals E M 3 and E M 5 in the symmetric meta -fragments seem to be different to the four orbitals E 1 – E 4 , but the orbitals E M 3 and E M 5 appear within the energy range from E 1 to E 4 despite the wider localization area, and in fact E M 3 and E M 5 show almost the same energy levels of E 2 and E 3 , respectively. 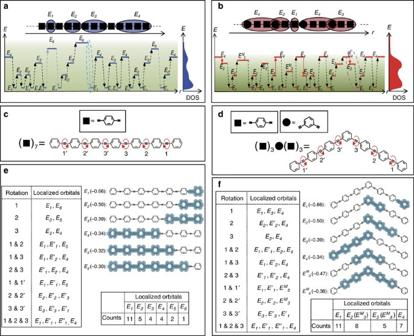Figure 1: Schematics of the orbital distribution and orbital localization in thepara- andmeta-junctioned wires. (a) Schematic of a wire of widely distributed localized molecular orbitals and its energy diagram for thepara-system. The blue elliptical regions indicate the non-zero amplitudes in each orbital,En, whereEnis a localized orbital in which the orbital amplitude is localized withinnunits. The position (r) in the energy diagram corresponds to the atomic/fragment position along the one-dimensional molecular wire. The horizontal bars (blue) in the energy diagram indicate the areas in which the orbital amplitudes have non-zero values. The dotted arrows are charge hopping processes, and the grey dotted arrows are the processes with large energy changes that are not included in themeta-junctioned system. (b) Schematic of a wire of narrowly distributed localized molecular orbitals and its energy diagram in themeta-junctioned system. The red elliptical regions indicate the non-zero amplitudes in each orbital,En. The horizontal bars (red) in the diagram indicate the areas with non-zero orbital amplitudes. The solid red arrows are fast hopping processes because of the orbital overlap. (c) Thepara-junctioned π-conjugated fragment. (d) Themeta-junctioned π-conjugated fragment. (e,f) The list of localized orbitals in thepara- andmeta-fragments by the rotations at positions 1 (1′), 2 (2′) and 3 (3′) shown inFig. 1cand the counts of each orbital present. The numbers in the parentheses are the orbital energies in the unit of hopping integral calculated using the simple Hückel model. The cyan circles indicate the non-zero orbital amplitudes. The orbitals with a prime or double prime,E′nandE′′n, indicate that the localization area is the same to that of the orbital without a prime,En. However, their position of localization is different fromEn. For example, the orbital amplitude ofE′1by Rotation 1 and 2 shown inFig. 1eis localized at the second benzene fragment from the right-hand edge. The orbital overlap at themeta-joint position in themeta-system can be easily confirmed (for example,E3andE4in Rotation 1). Figure 1a shows examples of energy level alignments in a 70-benzene unit based on the orbital counts. It is clear that the meta -system shows a narrower DOS than the para -system. In addition, in the para -system, a large energy change is required for one of the hopping processes (dotted circle in Fig. 1a ), corresponding to the case of Rotation 1, and this process becomes the rate-determining step. Such a slow step is not expected in the meta -system because Rotation 1 leads to the localized orbitals of E 1 and partially overlapped orbitals E 3 and E 4 (dotted circle in Fig. 1b ), and the rate-determining step is consequently the hopping process from E 3 to E 1 or E 4 to E 1 , the energy difference of which is smaller than the rate-determining step in the para -system ( E 6 to E 1 ). Therefore, the regularly localized molecular orbitals introduced by the meta -junctions are expected to be effective for high charge mobility. Figure 1: Schematics of the orbital distribution and orbital localization in the para - and meta -junctioned wires. ( a ) Schematic of a wire of widely distributed localized molecular orbitals and its energy diagram for the para -system. The blue elliptical regions indicate the non-zero amplitudes in each orbital, E n , where E n is a localized orbital in which the orbital amplitude is localized within n units. The position ( r ) in the energy diagram corresponds to the atomic/fragment position along the one-dimensional molecular wire. The horizontal bars (blue) in the energy diagram indicate the areas in which the orbital amplitudes have non-zero values. The dotted arrows are charge hopping processes, and the grey dotted arrows are the processes with large energy changes that are not included in the meta -junctioned system. ( b ) Schematic of a wire of narrowly distributed localized molecular orbitals and its energy diagram in the meta -junctioned system. The red elliptical regions indicate the non-zero amplitudes in each orbital, E n . The horizontal bars (red) in the diagram indicate the areas with non-zero orbital amplitudes. The solid red arrows are fast hopping processes because of the orbital overlap. ( c ) The para -junctioned π-conjugated fragment. ( d ) The meta -junctioned π-conjugated fragment. ( e , f ) The list of localized orbitals in the para - and meta -fragments by the rotations at positions 1 (1′), 2 (2′) and 3 (3′) shown in Fig. 1c and the counts of each orbital present. The numbers in the parentheses are the orbital energies in the unit of hopping integral calculated using the simple Hückel model. The cyan circles indicate the non-zero orbital amplitudes. The orbitals with a prime or double prime, E′ n and E′′ n , indicate that the localization area is the same to that of the orbital without a prime, E n . However, their position of localization is different from E n . For example, the orbital amplitude of E′ 1 by Rotation 1 and 2 shown in Fig. 1e is localized at the second benzene fragment from the right-hand edge. The orbital overlap at the meta -joint position in the meta- system can be easily confirmed (for example, E 3 and E 4 in Rotation 1). Full size image Preparation of linear and zigzag IMWs Meta -junctioned IMWs with an ideal molecular structure for achieving high charge mobilities were synthesized with the following characteristics: (1) a high coverage to isolate the π-conjugated chain, (2) tight insulation by narrow macrocycles to reduce structural fluctuation/deformation, (3) PE (phenylene-ethynylene) units of the same length in the para -segment, (4) perfect structural regularity with high symmetry and (5) high organic solubility for improved processability. To synthesize the desired molecular wires, linear and bent insulated OPE monomers with a high coverage ratio, structural regularity and organic solubility were prepared ( Fig. 2 ). The host–guest-linked compound 1 consists of permethylated α-cyclodextrin (CD) as an organic soluble cyclic host and a bis-PE unit as a π-conjugated guest [19] , [20] . The quantitative formation of the intramolecular self-inclusion complex 2 via hydrophilic and hydrophobic interactions of 1 in H 2 O/CH 3 OH (1:1) solution was confirmed by 1 H-NMR spectroscopy. A sequential Sonogashira cross-coupling reaction was then carried out between two molecules of 2 with para - or meta -diiodobenzene to yield linked and fixed [3]rotaxane monomers 3 and 4 , in which the inclusion state was maintained. The formation of 3 and 4 was confirmed by MALDI-TOF mass spectrometry and 2D NOESY NMR analysis ( Supplementary Fig. S8 ). Studies conducted using space-filling models revealed that the coverage ratio of the permethylated α-CD in the OPE unit of 3 was ~85%. The acetamide groups of 3 and 4 were then converted to iodo and then ethynyl groups to yield fixed [3]rotaxane monomers 5–8 containing the reactive site of the Sonogashira reaction at both ends. 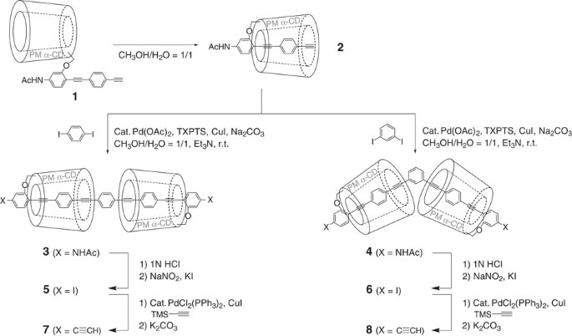Figure 2: Synthesis of linear and bent insulated OPE monomers 5–8. Complete experimental details and characterization are supplied in theSupplementary Methodssection. Figure 2: Synthesis of linear and bent insulated OPE monomers 5–8. Complete experimental details and characterization are supplied in the Supplementary Methods section. Full size image A defect-free linear IMW with a para -poly(phenylene–ethynylene) ( para -PPE) backbone was synthesized as a reference polymer via the Sonogashira copolymerization of 5 with 1,4-diethynylbenzene. Sonogashira copolymerization of 8 with 1,3-diiodobenzene yielded twisted IMW 10 containing three PE units between the meta -junctions ( Fig. 3 ). 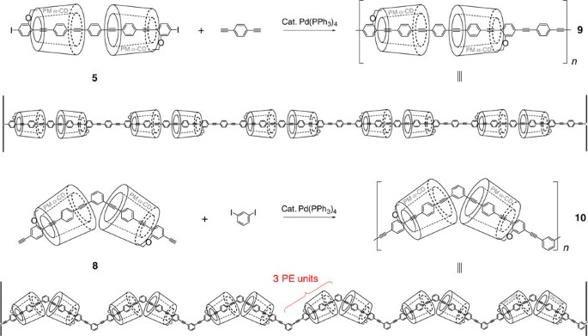Figure 3: Syntheses of linear and zigzag IMWs 9 and 10. Complete experimental details and characterization are supplied in theSupplementary Methodssection. Figure 3: Syntheses of linear and zigzag IMWs 9 and 10. Complete experimental details and characterization are supplied in the Supplementary Methods section. Full size image Measurements of intrinsic charge carrier mobility in IMWs Next, the potential for charge mobility of the prepared IMWs in the solid state was examined by simultaneously performing time-resolved microwave conductivity (TRMC) and transient absorption spectroscopy measurements [21] , [22] . The observed kinetic traces of the transient conductivity in solid films of 9 and 10 are shown in Fig. 4a . The para -PPE backbone in the linear IMW 9 exhibited effective photo-induced ionization upon excitation under ultraviolet exposure. This resulted in highly mobile positive holes (radical cations) on the backbones and stable scavenging of electrons by oxygen molecules. The kinetic traces of the transient absorption ascribed to the radical cations were evaluated quantitatively in their solid state using nano-second laser flash photolysis. Identical kinetic traces for the transient conductivity and optical absorption of the radical cations provided estimates of the intramolecular mobility of the holes on the backbone as μ ~0.75 cm 2 V −1 s −1 for the linear PE backbones stretched and locked tightly by the insulating clads of CD, as in 9 . 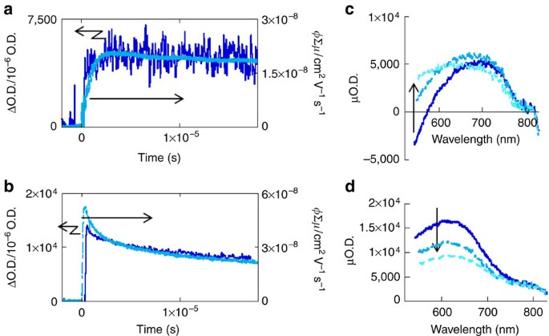Figure 4: Conductivity transients and transient absorption spectroscopy (TAS) of films of 9 and 10. (a,b) Conductivity transients observed upon excitation of 355 nm at 6.5–7.3 × 1015photons cm−2in cast films of9and10with kinetic traces at absorption maxima (690 nm for9and 630 nm for10) of the corresponding compounds. (c) TAS of a solid film of9upon exposure to 355 nm pulses at 5.0 × 1016photons cm−2recorded 2, 10 and 20 μs after excitation. (d) TAS of a solid film of10upon exposure to 355 nm pulses at 6.5 × 1016photons cm−2recorded at 2, 10 and 20 μs after excitation. Figure 4: Conductivity transients and transient absorption spectroscopy (TAS) of films of 9 and 10. ( a , b ) Conductivity transients observed upon excitation of 355 nm at 6.5–7.3 × 10 15 photons cm −2 in cast films of 9 and 10 with kinetic traces at absorption maxima (690 nm for 9 and 630 nm for 10 ) of the corresponding compounds. ( c ) TAS of a solid film of 9 upon exposure to 355 nm pulses at 5.0 × 10 16 photons cm −2 recorded 2, 10 and 20 μs after excitation. ( d ) TAS of a solid film of 10 upon exposure to 355 nm pulses at 6.5 × 10 16 photons cm −2 recorded at 2, 10 and 20 μs after excitation. Full size image The measured time constant of 2 × 10 6 s −1 , which is the signature of free carrier generation via a triplet–triplet annihilation scheme [23] , [24] , confirmed the photo-induced formation of charge carriers on the backbone of 9 . In contrast, rapid free carrier-formation processes are clearly overlapped for 10 . The contribution of the singlet excited states of 10 to the photo-carrier generation in these compounds is evident by tracing the transient absorption spectra and from the kinetics, as shown in Fig. 4b . Strong bleaching of the steady-state electronic absorption at 480 nm was nearly recovered within a time constant for the present transient absorption spectroscopy system of <10 ns, leading to a residual weak bleaching 2 μs after pulse excitation. Radical cations on the backbone of 10 appeared as a transient absorption band around 630 nm (ref. 10 ), indicating a nearly identical ratio (~1.8) to that of the molar extinction coefficients for the neutral and cationic states of 9 . It should be noted that, even in this time range, the kinetic traces for the conductivity and optical absorption transients are completely overlapped. This result suggests that different pathways via the triplet and singlet excited states effectively produce free positive charges on the conjugated backbone of 10 (ref. 25 ). The kinetic analysis also allows full experimental estimates of the charge carrier mobility on the backbones. Based on the value of the molar extinction coefficient for the steady-state of 10 per conjugation unit at 480 nm (3 × 10 5 cm −1 mol −1 dm 3 ), 10 +· ( ε 10 +· ) was estimated to be 5 × 10 5 cm −1 mol −1 dm 3 . This value provides a complete experimental estimate of the photo-carrier generation yield ( φ ), and hence, the value of the one-dimensional intramolecular mobility of the holes along the skeleton of 10 , of 2.1 cm 2 V −1 s −1 , which is the first time that intramolecular charge mobility above 1 cm 2 V −1 s −1 has been achieved as charge carrier hopping processes in π-conjugated polymers, with the mobility approaching the highest limit for the hopping transport of charge carriers. As expected, zigzag IMW 10 (2.1 cm 2 V −1 s −1 ) exhibited a higher intramolecular charge mobility than linear IMW 9 (0.75 cm 2 V −1 s −1 ). This value was approximately twice that of an insulated polythiophene (0.9 cm 2 V −1 s −1 ) (ref. 26 ) and a ladder porphyrin polymer (0.93 cm 2 V −1 s −1 ) (ref. 27 ). Theoretical study on the model systems To elucidate the mechanism of the higher charge mobility in the zigzag IMW, quantum wave-packet scattering simulations [28] , [29] were carried out for the zigzag and linear wires. Because the original IMWs include CD molecules, which are not favourable for calculations, we propose an effective IMW (e-IMW) model based on the theoretical finding that the rotation barrier of a benzene in the CD-covered wire at room temperature (RT) is almost equal to that in the uncovered wire at 60 K [30] (see Supplementary Note 3 ). That is, we can estimate the wire dynamics of IMWs at RT from those of an uncovered wire (e-IMW) at 60 K. This fact in turn corresponds to the reduced structural fluctuation/deformation of IMWs, the second characteristic of IMWs. The transport mechanism in the zigzag and linear IMWs is considered to be a mixture of the coherent, incoherent and diffusive regions of the quantum transport, and thus a wave-packet scattering method was adopted that can represent quantum transport in those regions. Wave-packet simulations were carried out as follows: (1) First-principles molecular dynamics calculations of the one-dimensional e-IMWs were carried out to determine the molecular configurations as a function of time; (2) The time-dependent Hamiltonian matrices in the π-orbital approximation were obtained from the configurations; (3) Wave-packet simulations were carried out using the time-dependent Schrödinger equation based on the time-dependent Hamiltonian; and (4) The mean-square displacements (MSDs), r 2 ( t )− r ( t ) 2 ≡ r ( t ) 2 , and diffusion coefficients were calculated from the scattered (that is, propagated) wave packet as , and the charge mobility was obtained using the Einstein relationship ( μ = De / k B T ) for both systems, where r , t , k B and T are the position vector, simulation time, Boltzmann constant and temperature, respectively. The expected value of position r ( t ) can be calculated using the wave packet ψ( t ) as ψ( t )| r ( t )|ψ( t ) . Meta -junctioned systems in which a single meta -joint appears per three PE units (abbreviated as meta(3) ) were used as the first target (see Fig. 1d ). The computational details in the wave-packet scattering simulations are the same as those described in our previous study [29] , and the computational conditions for the first-principles molecular dynamics calculations and time-dependent Hamiltonian are described in Supplementary Figs S10 and S11 . 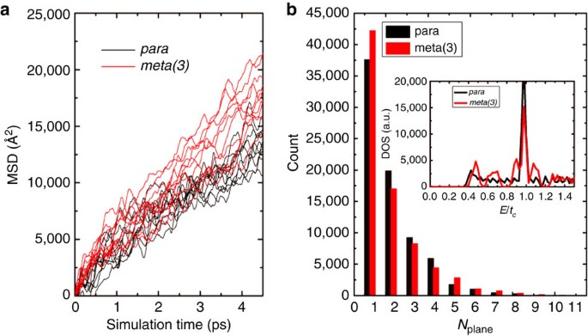Figure 5: Calculated MSDs and length histograms of the planar segments. (a) MSDs for 10 typical out of configurations for both theparaandmeta(3)systems. (b) Length histograms of the planar segments in theparaandmeta(3)systems.Nplaneis the number of benzene rings within a planar segment. The inset shows the time-averaged DOSs. In these simulations, a wave-packet energy of 0.5tcand a half-width of 0.015tcwere used as the incoming wave packet, which corresponds to the experimental conditions for light irradiation with an energy of 2.5 eV, becausetcis nearly equal to 2.5 eV in carbon systems. Figure 5a shows the typical calculated MSDs of the para and meta(3) systems. The MSDs depend on the wire configurations; for instance, the wave-packet diffusion within a planar structure is faster than that in a non-planar structure. The meta(3) system was found to have much larger MSDs than the para -system. The average values of the mobilities for the para and meta(3) systems were calculated to be 5.4±1.4 and 7.2±2.0 cm 2 V −1 s −1 , respectively. Although the calculated mobilities of the para and meta(3) systems are quantitatively larger than the observed ones, the qualitative relationship of the mobilities for both systems is the same. Figure 5: Calculated MSDs and length histograms of the planar segments. ( a ) MSDs for 10 typical out of configurations for both the para and meta(3) systems. ( b ) Length histograms of the planar segments in the para and meta(3) systems. N plane is the number of benzene rings within a planar segment. The inset shows the time-averaged DOSs. In these simulations, a wave-packet energy of 0.5 t c and a half-width of 0.015 t c were used as the incoming wave packet, which corresponds to the experimental conditions for light irradiation with an energy of 2.5 eV, because t c is nearly equal to 2.5 eV in carbon systems. Full size image Figure 5b shows the length histograms of the sequential planar segments in the para and meta(3) systems; the neighbouring benzene rings with dihedral angles in the range from −10° to 10° were regarded as a sequential planar segment. Although the histogram indicates a difference in the flatness between the para and meta(3) systems, it cannot be concluded whether the difference in the flatness is the dominant reason for the higher mobility in the meta(3) system. To clarify this point, wave-packet calculations of a modified- meta(3) system using the dihedral angles of the para system were carried out. That is, the only difference between the modified- meta(3) and para systems is the connectivity between the benzene fragments. From the calculated MSDs for the modified- meta(3) , an average mobility of 7.2±2.2 cm 2 V −1 s −1 was obtained, which is nearly equal to that of the original meta(3) system. Thus, the main reason for the higher mobility in the meta(3) system is not structural planarity but connectivity (that is, meta -joint); the meta -connectivity in turn results in orbitals with a narrower DOS than the para -system orbitals. This is shown in the inset of Fig. 5b ; the time-averaged DOS spreads across the region from 0.4 to 1.4 t c in the para -system, whereas it splits into several groups in the meta -system. Therefore, the meta -connectivity is essential for generating the regularly localized orbitals that accelerate the charge hopping process. Another point of interest is the dependence on para- length of the mobility in the meta -systems. To examine the effect of elongation of the length of the para -segments, zigzag IMWs 11 and 12 containing six and ten PE units between the meta -junctions, respectively, were synthesized ( Fig. 6 ) via Sonogashira copolymerization of 5 with 1,3-diethynylbenzene (to prepare 11 ) and 7 with 6 (to prepare 12 ). Notably, when the length between the para -segments of the IMWs 10 was increased from three ( 10 ) to ten ( 12 ) PE units, the intramolecular charge mobility increased to 8.5 cm 2 V −1 s −1 ( Supplementary Fig. S11 ). In general, the cross-boundaries for the hopping and band transport of charge carriers occur when the mobility is in the range 1–10 cm 2 V −1 s −1 , and thus the value obtained here nearly reaches the highest limit for the mobility of charge carriers transported via inter-site hopping processes. The temperature dependence of the transient photoconductivity was also examined for 12 ( Supplementary Fig. S12 ). The Arrhenius plot was found to have a slope with a low activation energy of 20 meV at 1/ T <0.0035, even though a slightly higher energy of 40 meV was observed over the entire temperature range. The energy at the higher temperatures, which was almost equivalent to the thermal energy of electrons, strongly suggests that the charge carrier mobility occurs on the conjugated backbone of 12 in the cross-boundary range for charge carrier transport mechanisms. A much higher value of mobility, 600 cm 2 V −1 s −1 , has previously been reported, defined as an intramolecular mobility in the electronic band-conduction model, where the phonon scattering of the charge carriers has a negative effect on the overall transport of the charge carriers [16] . In the present work, hopping transport is the predominant process and 8.5 cm 2 V −1 s −1 is the highest mobility value for the one-dimensional intramolecular hopping of holes along a π-conjugated polymer reported thus far [25] . 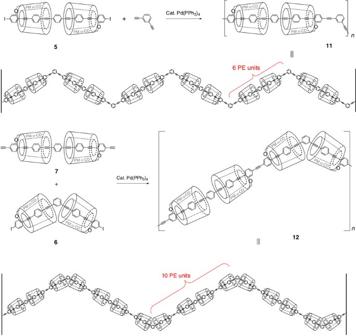Figure 6: Syntheses of zigzag IMWs 11 and 12 with elongatedpara-segments between themeta-junctions. Complete experimental details and characterization are supplied in theSupplementary Methodssection. With an electric field strength of E =25 V cm −1 used in the microwave cavity, the mean local displacement of charge carriers, dx , can be estimated as follows: Figure 6: Syntheses of zigzag IMWs 11 and 12 with elongated para -segments between the meta -junctions. Complete experimental details and characterization are supplied in the Supplementary Methods section. Full size image where ω is the frequency of microwaves (9.1 GHz) and Q is the Q -value (~2,500) of the cavity representing the average number of interactions between a charge carrier and microwave in the cavity. The derived value of dx was estimated to be in the range 4–12 nm along the backbone of 12 , with the temperature increasing from 210 to 380 K, which is larger than the inter-site distance in the backbone of 12 at the higher temperature; however, it is of the same order of magnitude to the distance at the lower temperature. The increasing activation energy (up to 40 meV), which overcomes the thermal energy of electrons at the lower temperature range, produces a constrained charge carrier at a hopping site, and hence, lowers the contribution from inter-site hopping processes to the conductivity transients [31] . This is in good agreement with the equivalent dx in the temperature range below 280 K. The estimated dx value corresponds well to the theoretically calculated localization length of ~14 nm, as shown in Supplementary Note 4 . In addition, the first-principles free energy calculations at the level of the single-configuration interaction with the 6–31 G basis set revealed that the activation barrier of benzene rotation leading to orbital localization (that is, charge hopping) is in the range 39–154 meV, which also corresponds to the experimentally determined activation barrier ( Supplementary Note 5 ). The MSDs and mobilities of the meta(6) and meta(10) systems were calculated using the same computational procedures adopted in the para and meta(3) cases. The calculated mobilities of the meta(6) and meta(10) systems are 9.5±1.3 and 14.0±5.0 cm 2 V −1 s −1 , respectively. The computational results qualitatively agree well with the observed results. On analysing the structural configurations of the meta(6) and meta(10) systems by plotting length histograms of the planar segments (not shown), it was found that the degree of flatness of the para -segments between the meta -joints meta(6) and meta(10) is higher than that of the para -junctioned system. The flatness of the meta -junctioned systems is high in the order meta(10) > meta(6) > meta(3) . Thus, in the meta -junctioned systems, improvement of the flatness has an important role in the enhancement of the charge mobility, and the longer para -segments also work well for the enhancement of the charge mobility via a coherent charge transport process. In conclusion, we have synthesized structurally defined IMWs with linear and zigzag PPE backbone units via Sonogashira copolymerization of linear and bent insulated OPE monomers with a fixed [3]rotaxane structure. Complete contactless measurement of the intramolecular mobility revealed the formation of a highly insulated organic semiconductor wire with extremely high hole mobility by simply changing the configuration of polymer chain from linear to zigzag. This high mobility was achieved by regularly localizing the π-molecular orbitals to equalize the distance and orbital level between the hopping sites. Interestingly, the intramolecular charge mobility increased to 8.5 cm 2 V −1 s −1 by increasing the length of the insulated PE units between the meta -segments of the zigzag IMWs. This value in the cross-boundary range of hopping, and band transport is comparable to the highest value in amorphous silicon [32] , [33] . Moreover, even in the solid state, it is the highest value for effective hopping transport of holes along one-dimensional molecular wires, including polysilicons (0.23 cm 2 V −1 s −1 ) [21] . This suggests that this design concept provides highly effective pathways for inter-site hopping processes with well-balanced inter-site activation energies and thermal energy of mobile charge carriers on the conjugated skeleton. In addition, according to the theoretical analysis, we confirmed that the molecular properties designed using this principle work well for obtaining ideal charge mobility in π-conjugated polymer chains. Further studies are being planned for investigation of the optimal length of the insulated para -segments. Synthesis of IMWs Host–guest-linked bis-PE 1 was prepared by the procedure reported previously [19] . Other reagents were purchased from commercial sources and used without further purification. A detailed description of insulated OPE monomers synthesis can be found in Supplementary Methods . All IMWs were synthesized by Sonogashira coupling of insulated OPE monomer with coupling partner in the presence of Pd(0) catalyst. High-molecular-weight IMWs were separated by preparative recycling gel permeation chromatography. First-principles calculations The unit cell of the meta- and para -junctioned one-dimensional periodic systems includes 12 benzene fragments. The cell parameters and initial structures for each system were determined using the first-principles density functional code SIESTA [34] . The density functional and basis set used in this study are the generalized gradient approximation with the Perdew, Burke and Ernzerhof [35] functional and single zeta polarization. For the first-principles molecular dynamics, a time step of 1.0 fs and temperature of 60 K were used, and wire structures after equilibration (5,000 steps) for 5 ps were used in wave-packet calculations. Flash-photolysis TRMC measurement In a microwave circuit, a resonant cavity with Q -value of 2,500 was used to preserve a high degree of sensitivity in the measurement of conductivity. The resonant frequency and the microwave power were set at ~9.1 GHz and 3 mW, respectively. Third harmonic generation (355 nm) of a Nd:YAG laser (Spectra-Physics Inc., INDI-HG, 4 ns FWHM, λ ex =355 nm, 5 mJ per pulse) was used as an excitation source. The TRMC signal from a diode was recorded on a digital oscilloscope (TDS 3032B; Tektronix). Polymers were casted onto quartz substrate from toluene solution at 3 wt% concentration and dried under vacuum for 1 h. The transmittance of the films were measured by a JASCO V-570 spectrophotometer, and also confirmed by a PE25 power meter of Ophir Optoronics Ltd. for the laser light excitation. Transient absorption measurement Time-dependent absorption spectral changes were monitored by Hamamatsu C7700 streak camera via a Hamamatsu C5094 spectrometer upon direct excitation of the identical solid-state polymer films used for TRMC measurements using a third harmonic generation ( λ =355 nm) light pulses from the Nd:YAG laser. To correct a two-dimensional time-wavelength correlation data of the transient absorption, the streak scope images were averaged over 1,600 images via a high speed camera (Hamamatsu C4742-95). Impurity effects A solution of IMWs 9 , 10 , 11 and 12 was stirred with QuadraSil TA silica-supported metal scavenger (Aldrich) at RT for 18 h. After filtration and evaporation of the solvent, the product was analysed with respect to palladium content by using inductively coupled plasma mass spectrometry. We found that these IMWs only contained <550 p.p.m. of palladium impurities after this scavenging process. The aggregates of metal residue in the polymerization reactions contribute to the conductivity transients monitored by TRMC, and the effects have been traced quantitatively by adding Pd catalyst and the other metal aggregates and nanoparticle into the solid-state conjugated polymer systems [36] , [37] . The significant contribution from the charge carrier trapping on metal aggregates was observed for addition of Pd catalyst in the concentration range ~1–5 wt% with a decrease in the transient conductivity signals [36] . Thus, the increase in the conductivity signal due to the local motion of charge carriers on Au nanoparticles in the conjugated polymer composites containing over 5 wt% Au nanoparticles was monitored [37] . This strongly indicates the negligible effects of the residual Pd catalysts in the conductivity transient observed for the present conjugated polymer systems. How to cite this article: Terao, J. et al . Design principle for increasing charge mobility of π-conjugated polymers using regularly localized molecular orbitals. Nat. Commun. 4:1691 doi: 10.1038/ncomms2707 (2013).